The highly conserved domain of unknown function 1792 has a distinct glycosyltransferase fold More than 33,000 glycosyltransferases have been identified. Structural studies, however, have only revealed two distinct glycosyltransferase (GT) folds, GT-A and GT-B. Here we report a 1.34-Å resolution X-ray crystallographic structure of a previously uncharacterized ‘domain of unknown function’ 1792 (DUF1792) and show that the domain adopts a new fold and is required for glycosylation of a family of serine-rich repeat streptococcal adhesins. Biochemical studies reveal that the domain is a glucosyltransferase, and it catalyses the transfer of glucose to the branch point of the hexasaccharide O-linked to the serine-rich repeat of the bacterial adhesin, Fap1 of Streptococcus parasanguinis . DUF1792 homologues from both Gram-positive and Gram-negative bacteria also exhibit the activity. Thus, DUF1792 represents a new family of glycosyltransferases; therefore, we designate it as a GT-D glycosyltransferase fold. As the domain is highly conserved in bacteria and not found in eukaryotes, it can be explored as a new antibacterial target. Protein glycosylation, catalysed by glycosyltransferases, is an important protein modification found in both prokaryotes [1] and eukaryotes [2] where it plays crucial roles in cell–cell recognition, adhesion and intracellular sorting [3] , [4] , [5] . Since the classification system for glycosyltransferases based on amino-acid sequence similarity was proposed by Campbell et al. in 1997 (ref. 6) [6] , the number of glycosyltransferases has grown enormously to over 33,000, organized into over 100 subfamilies [6] , [7] , [8] . In contrast, numerous structural studies have revealed that the structural folds displayed by this large number of glycosyltransferases are limited and only two distinct structural folds, GT-A and GT-B, have been rigorously characterized [9] , [10] . GT-A displays a single Rossmann fold (topology β/α/β/α/β) and a conserved ‘DXD’ metal-binding motif [11] , [12] . In contrast, GT-B possesses twin Rossmann folds that face each other and are linked flexibly by the active site within the resulting cleft [13] , [14] . In contrast, this family does not require metal ions for its activity. There is another previously named glycosyltransferase fold, the GT-C fold. Recent structural studies of two predicted GT-C types of enzymes (oligosaccharyltransferase STT3 (ref. 15 ) and peptidoglycan synthesizing glycosyltransferase PBP2 (refs 16 , 17 )) suggest that they actually adopt different protein folds. Thus, whether GT-C represents a distinct glycosyltransferase fold remains controversial. Serine-rich repeat glycoproteins (SRRPs) are a growing family of bacterial adhesins and they play important roles in bacterial fitness and virulence [18] , [19] , [20] . Fimbriae-associated protein (Fap1) was the first SRRP-identified protein [21] . It is heavily O-glycosylated by Glc-GlcNAc-linked oligosaccharides containing up to four additional sugars [22] . Fap1 modulates bacterial biofilm formation in the oral bacterium Streptococcus parasanguinis [23] . Fap1-like SRRPs have since been identified from other streptococci [24] , [25] , [26] , staphylococci [27] , [28] , [29] and other Gram-positive bacteria [30] . Biogenesis of Fap1 in S. parasanguinis is controlled by a gene cluster adjacent to this SRRP structural gene [22] . Analogous gene clusters are highly conserved in streptococci and staphylococci [30] . Glycosylation and secretion of Fap1 is mediated by 11 genes. A gene cluster coding for four putative glycosyltransferases, Gly, Gtf3, GalT1 and GalT2 is located upstream of fap1 , and another gene cluster producing accessory secretion components, SecY2, SecA2, Gap1, Gap2 and Gap3, and two putative glycosyltransferases (Gtf1 and Gtf2) are located downstream of fap1 (refs 31 , 32 ). Gtf1 and Gtf2 form a protein complex that catalyses the first step of glycosylation by transferring GlcNAc residues to the Fap1 polypeptide [31] , [33] , [34] , while Gtf3 catalyses the second step of glycosylation by transferring Glc residues to the GlcNAc-modified Fap1 (refs 35 , 36 ). However, it is not yet known which enzymes mediate the subsequent glycosylation steps. GalT1 in the fap1 locus was annotated as a glycosyltransferase since the C terminus of GalT1 is predicted to have a classic GT-A fold and shares significant homology with galactosyltransferases. A domain of unknown function is found at the N terminus of GalT1, which belongs to an uncharacterized DUF1792 superfamily (cl07392: DUF1792 Superfamily, commonly found at the C terminus of proteins that also contain the glycosyltransferase domain at the N terminus). DUF1792 is highly conserved in numerous glycosyltransferases that have the same organization as exhibited in GalT1, and the DUF1792 domain module also exists by itself in streptococci, lactobacilli [37] and even Gram-negative bacteria [38] . Sequence analysis and structural prediction reveal that DUF1792 does not share any homology with known glycosyltransferases, suggesting that it represents a new domain that may possess a unique activity. In this study, we determine the glycan sequence on Fap1 and demonstrate that DUF1792 is a novel glucosyltransferase that catalyses the third step of Fap1 glycosylation. Moreover, a 1.34-Å resolution X-ray crystal structure of DUF1792 has revealed that DUF1792 is structurally distinct from all known GT folds of glycosyltransferases and contains a new metal-binding site. The glycosyltransferase activity of DUF1792 appears to be highly conserved in pathogenic streptococci and fusobacteria. We conclude that DUF1792 represents a highly conserved glycosyltransferase superfamily with a novel GT fold and we designate this new glycosyltransferase fold as a GT-D type. Characterization of the O-glycans on Fap1 We employed a variety of mass spectrometric glycomic strategies to characterize Fap1 glycosylation. As it was difficult to isolate native Fap1 in sufficient quantities for in-depth structure analysis, we first characterized the glycosylation of recombinant Fap1 that we obtained by co-expression of recombinant Fap1 (rFap1) [35] with all the glycosyltransferases identified from the fap1 locus. rFap1 was purified and subjected to beta-elimination to release the O-linked glycans for MS analysis. Matrix-assisted laser desorption/ionization–time of flight (MALDI–TOF) mass fingerprinting ( Fig. 1a,b ) of the beta-eliminated permethylated glycans showed a mixture of glycans ranging in size from a monosaccharide (HexNAc) up to a hexasaccharide comprising one deoxyhexose, two HexNAcs and three hexoses. The latter is consistent with a previously reported monosaccharide composition for the native Fap1 glycan [22] . The smaller glycans correspond to biosynthetic precursors. Each peak from the glycan fingerprint was further analysed by MALDI–TOF/TOF to generate glycan sequences. The MS/MS spectrum of the hexasaccharide peak at m/z 1,361.6 is shown in Fig. 1c . The data are fully consistent with the branched structure shown in the cartoon annotation on this figure. The identities of the sugars and their linkages were determined by additional GC-EI-MS experiments. 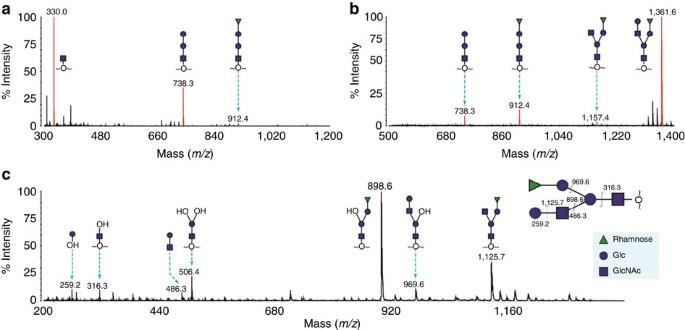Figure 1: Mass spectrometric analysis of rFap1 glycan. The glycans were reductively eliminated from the protein, and permethylated. Derivatized glycans were purified on reverse phase C18 Sep-Pak columns. The MALDI–TOF spectra of the 35% acetonitrile (MeCN) eluate (a), the 50% MeCN eluate (b) and MALDI–TOF/TOF spectrum of the peak at mass-to-charge ratio (m/z) 1,361.6 (c) are shown. In spectra (a,b), peaks corresponding to sodiated glycans are coloured red and annotated withm/zand glycan structures. Other black signals are due to under-permethylation (minus 14 inm/z) or contaminations from the matrix. In spectrac, peaks corresponding to diagnostic fragments are annotated withm/zand glycan structure. Notably, the peak atm/z506.4 corresponds to a double-cleaved fragment, indicating that the fully synthesized glycan is branched. Sugar linkage analysis of partially methylated alditol acetates ( Supplementary Table 1 ) determined rhamnose and glucose as non-reducing sugars in the hexasaccharide, and identified the reducing sugar as 6-linked GlcNAc. Other linkages observed were 3-linked GlcNAc, and 3- and 2,6-linked Glc, the latter being consistent with the branched sequence shown in Fig. 1c . Figure 1: Mass spectrometric analysis of rFap1 glycan. The glycans were reductively eliminated from the protein, and permethylated. Derivatized glycans were purified on reverse phase C18 Sep-Pak columns. The MALDI–TOF spectra of the 35% acetonitrile (MeCN) eluate ( a ), the 50% MeCN eluate ( b ) and MALDI–TOF/TOF spectrum of the peak at mass-to-charge ratio ( m/z ) 1,361.6 ( c ) are shown. In spectra ( a , b ), peaks corresponding to sodiated glycans are coloured red and annotated with m/z and glycan structures. Other black signals are due to under-permethylation (minus 14 in m/z ) or contaminations from the matrix. In spectra c , peaks corresponding to diagnostic fragments are annotated with m/z and glycan structure. Notably, the peak at m/z 506.4 corresponds to a double-cleaved fragment, indicating that the fully synthesized glycan is branched. Full size image Collectively, the glycomics data show that the largest Fap1 glycan has the sequence Rha1-3Glc1-(Glc1-3GlcNAc1-)2,6Glc1-6GlcNAc. Moreover, the absence of a disaccharide intermediate in the glycomic fingerprints ( Fig. 1a,b ) suggests that there is a rapid incorporation of the second glucose in the biosynthetic pathway leading to the hexasaccharide. In addition, since the same glycan fingerprint was observed in the native Fap1 purified from S. parasanguinis ( Supplementary Fig. 1 ), we conclude that the latter shares the O-glycan sequences identified in our in-depth studies of recombinant samples. DUF1792 is required for the third step of Fap1 glycosylation While we have determined the first two steps of Fap1 glycosylation [34] , [36] the remaining glycosylation steps are unknown. In a search for proteins responsible for the subsequent steps of Fap1 glycosylation we identified dGT1 (previously named GalT1 because of its annotated function; we rename it as dGT1 as it has two functional domains). dGT1 is predicted to be a glycosyltransferase since it possesses a putative GT-A-type glycosyltransferase domain at the C terminus. Interestingly, dGT1 also contains a distinct domain of unknown function DUF1792 at the N terminus ( Fig. 2a ). In vitro glycosylation assays revealed that full-length dGT1 has a glucosyltransferase activity, transferring glucose residues to Glc-GlcNAc-modified Fap1 ( Fig. 2b ), suggesting dGT1 is involved in the third step of Fap1 glycosylation. To dissect the individual dGT1 domain(s) involved, we expressed both the N-terminal DUF1792 domain (amino acids 1–272) and the C-terminal domain (amino acids 273–582), and determined their activity. Unexpectedly, the N-terminal DUF1792 domain, but not the predicted C-terminal glycosyltransferase GT-A domain, is responsible for the in vitro glucosyltransferase activity ( Fig. 2b ). Moreover, the glucosyltransferase activity of DUF1792 is dependent on the presence of metal ions ( Fig. 2c ). Mn 2+ maximized the activity. However, DUF1792 does not have the classic metal-binding motif, DXD, found in GT-A family of glycosyltransferases, suggesting that DUF1792 represents a new type of glycosyltransferase. 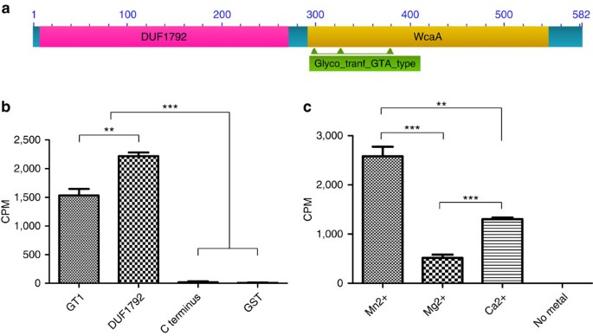Figure 2: Glycosyltransferase activity of DUF1792. (a) Diagram of dGT1. dGT1 consists of two domains: an N-terminal DUF1792 and a C-terminal GT-A-like domain (WcaA, glycosyltransferase involved in cell wall biosynthesis). (b)In vitroglycosyltransferase activity of DUF1792. Purified dGlT1, and N-terminal DUF1792 fusion proteins catalysed the transfer of3H-labelled glucose from an activated donor sugar, UDP-3H glucose to Gtf1/2, 3-modified Fap1 inin vitroglycosylation reactions, while the C terminus of dGT1 GST fusion protein and GST failed to transfer. Heated inactivated proteins were used as negative controls to normalize the transfer activity by CPM. (c) Metal ions are required for glycosyltransferase activity of DUF1792. Divalent metal ions, Mn2+, Mg2+and Ca2+(10 mM), promoted the transfer of3H-labelled glucose from an activated donor sugar, UDP-3H glucose to Gtf1/2, 3-modified Fap1 inin vitroglycosylation reactions. The values obtained from three different experiments represent means±s.e.m.’s. Significant differences were indicated by asterisks (**P<0.01, ***P<0.001). Figure 2: Glycosyltransferase activity of DUF1792. ( a ) Diagram of dGT1. dGT1 consists of two domains: an N-terminal DUF1792 and a C-terminal GT-A-like domain (WcaA, glycosyltransferase involved in cell wall biosynthesis). ( b ) In vitro glycosyltransferase activity of DUF1792. Purified dGlT1, and N-terminal DUF1792 fusion proteins catalysed the transfer of 3 H-labelled glucose from an activated donor sugar, UDP- 3 H glucose to Gtf1/2, 3-modified Fap1 in in vitro glycosylation reactions, while the C terminus of dGT1 GST fusion protein and GST failed to transfer. Heated inactivated proteins were used as negative controls to normalize the transfer activity by CPM. ( c ) Metal ions are required for glycosyltransferase activity of DUF1792. Divalent metal ions, Mn 2+ , Mg 2+ and Ca2 + (10 mM), promoted the transfer of 3 H-labelled glucose from an activated donor sugar, UDP- 3 H glucose to Gtf1/2, 3-modified Fap1 in in vitro glycosylation reactions. The values obtained from three different experiments represent means±s.e.m.’s. Significant differences were indicated by asterisks (** P <0.01, *** P <0.001). Full size image To further define the function of DUF1792, we examined the ability of DUF1792 to catalyse the third step of Fap1 glycosylation using a well-established Escherichia coli glycosylation system [35] . Since we have demonstrated that Gtf1/2 and Gtf3 catalyse the first two steps of Fap1 glycosylation, respectively, we co-expressed either DUF1792 or the full-length dGT1 with Gtf1/2, 3 and recombinant Fap1 (rFap1) [35] to determine whether dGT1 or DUF1792 further glycosylates the Gtf1/2, 3-modified rFap1. Indeed, dGT1 retarded the migration of the Gtf1/2, 3-modified rFap1 ( Fig. 3a , lane 3 versus 2), suggesting additional modification by dGT1. Interestingly, the migration of the modified rFap1 was further retarded when co-expressed with the DUF1792 domain itself ( Fig. 3a , lane 4). This is also true for the in vitro glycosyltransferase activity ( Fig. 2b ). The activity of DUF1792 is consistently higher than that from the full-length dGT1, suggesting the dGT1 C terminus may have an additional unknown glycosyltransferase activity that coordinates with the function of DUF1792 in vitro . To further determine the relative contribution of DUF1792 and C-terminal dGT1 to Fap1 glycosylation in the native host S. parasanguinis , the dGT1 mutant of S. parasanguinis was complemented by either DUF1792 or C-terminal dGT1, and then examined by Fap1-specific antibody mAbE42. The DUF1792 alone significantly retarded the migration of Fap1 indicative of glycosylation ( Fig. 3b , lane 5) in comparison with the dGT1 mutant ( Fig. 3b , lane 3), albeit it did not restore the migration as the full-length dGT1 ( Fig. 3b , lane 4). By contrast, the C-terminal dGT1 failed to restore the migration, suggesting that the DUF1792 domain is more important than the C-terminal domain in vivo in S. parasanguinis , and that both domains are required for biogenesis of mature Fap1. The detailed function of the C-terminal domain and how it contributes to the Fap1 glycosylation is under active investigation. DUF1792 is highly conserved in streptococci and several Gram-negative bacteria ( Fig. 3c and Supplementary Fig. 2 ). It is also present in archea ( Supplementary Fig. 2 ). To assess the functional conservation of DUF1792, we selected DUF1792 homologues from other streptococci and a Gram-negative bacterium Fusobacterium nucleatum to evaluate whether they can further modify the Fap1 glycosylated by Gtf1/2, 3. All DUF1792 homologues ( Fig. 3a , lanes 5–9 versus 2) retarded the migration of the Gtf123-modified Fap1, suggesting that additional sugar residues were transferred to the Gtf123-modified Fap1. 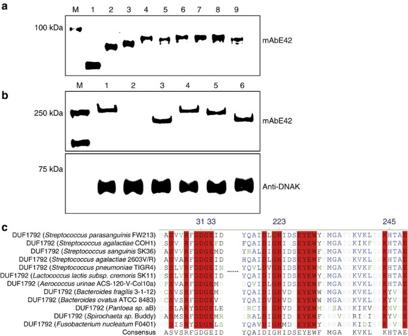Figure 3: The glycosyltransferase activity, DXE motif, and UDP binding domain of DUF1792 are conserved. (a) DUF1792 is functionally conserved. DUF1792 homologues from a variety of bacterial species were cloned into vector pGEx-6p-1 and co-transformed inE. colicarrying rFap1 and Gtf1/2, 3 to determine the ability of DUF1792 to catalyse the transfer of additional sugar residues to Gtf1/2, 3-modified rFap1. Cell lysates from rFap1 (1), Gtf1/2, 3-modified rFap1 (2) and Gtf1/2, 3-modified rFap1 coexpressed with dGT1 ofS. parasanguinis(3), or with DUF1792 fromS. parasanguinis(4),S. agalactiaeCOH1 (5);S. sanguinisSK36 (6),S. agalactiae2603 V/R (7),S. pneumoniaeTIGR4 (8) andF. nucleatumF0401 (9) were subjected to western blot analysis with Fap1-specific antibody E42. All DUF1792 homologues retarded the migration of rFap1, suggesting that they promoted the transfer of additional sugar residues to Gtf1/2, 3-modified Fap1. (b) Contribution of DUF1792 to glycosylation of Fap1. Wild-type dGT1, N-terminal dGT1-DUF1792, C-terminal dGT1 constructs were used to complement the dGT1mutant inS. parasanguinis. Cell lysates from wild-typeS. parasanguinis(1); Fap1 mutant (2); dGT1 mutant (3); the dGT1mutant complemented with the dGT1full-length gene (4), DUF1792 (5); and C-terminal dGT1 (6) were subjected to western blot analysis with Fap1-peptide-specific mAbE42 (top) and anti-DNAK antibody (bottom) as a sample loading control. Complementation of DUF1792 produces an intermediate of Fap1, while the complementation with the C terminus alone has the same phenotype as dGT1 mutant. (c)The DXE motif and UDP-binding sites are highly conserved in bacteria. DUF1792 homologues were identified from a group of streptococci,Lactobacillus lactisand several Gram-negative bacteria. The regions flanking the DGE motif and UDP-binding sites were compared. The invariant amino-acid residues highlighted in red and consensus sequence was deduced. Figure 3: The glycosyltransferase activity, DXE motif, and UDP binding domain of DUF1792 are conserved. ( a ) DUF1792 is functionally conserved. DUF1792 homologues from a variety of bacterial species were cloned into vector pGEx-6p-1 and co-transformed in E. coli carrying rFap1 and Gtf1/2, 3 to determine the ability of DUF1792 to catalyse the transfer of additional sugar residues to Gtf1/2, 3-modified rFap1. Cell lysates from rFap1 (1), Gtf1/2, 3-modified rFap1 (2) and Gtf1/2, 3-modified rFap1 coexpressed with dGT1 of S. parasanguinis (3), or with DUF1792 from S. parasanguinis (4), S. agalactiae COH1 (5); S. sanguinis SK36 (6), S. agalactiae 2603 V/R (7), S. pneumoniae TIGR4 (8) and F. nucleatum F0401 (9) were subjected to western blot analysis with Fap1-specific antibody E42. All DUF1792 homologues retarded the migration of rFap1, suggesting that they promoted the transfer of additional sugar residues to Gtf1/2, 3-modified Fap1. ( b ) Contribution of DUF1792 to glycosylation of Fap1. Wild-type dGT1, N-terminal dGT1-DUF1792, C-terminal dGT1 constructs were used to complement the d GT1 mutant in S. parasanguinis . Cell lysates from wild-type S. parasanguinis (1); Fap1 mutant (2); dGT1 mutant (3); the d GT1 mutant complemented with the d GT1 full-length gene (4), DUF1792 (5); and C-terminal dGT1 (6) were subjected to western blot analysis with Fap1-peptide-specific mAbE42 (top) and anti-DNAK antibody (bottom) as a sample loading control. Complementation of DUF1792 produces an intermediate of Fap1, while the complementation with the C terminus alone has the same phenotype as dGT1 mutant. ( c )The DXE motif and UDP-binding sites are highly conserved in bacteria. DUF1792 homologues were identified from a group of streptococci, Lactobacillus lactis and several Gram-negative bacteria. The regions flanking the DGE motif and UDP-binding sites were compared. The invariant amino-acid residues highlighted in red and consensus sequence was deduced. Full size image To further confirm that DUF1792 is capable of transferring Glc to the Glc-GlcNAc-modified Fap1 revealed by in vitro glycosylation assays ( Fig. 2b,c ), we performed glycan profiling analysis. In the presence of DUF1792, the glycan mass of this recombinant Fap1 increased by a hexose increment (compare Fig. 4a,b ), indicative of addition of Glc to the Glc-GlcNAc-modified Fap1. Since sugar and linkage analyses (see above) established that the only hexose contained in rFap1 glycan is glucose, it is reasonable to deduce that DUF1792 has a glucosyltransferase activity. Moreover, by exploiting a glycomics strategy incorporating MS fingerprinting of peracetylated derivatives before and after chromium trioxide oxidation [39] , we showed that DUF1792 attaches the glucose in a beta anomeric linkage. Under the oxidation conditions employed, alpha-linked peracetylated sugars are resistant to oxidation, while beta-linked sugars are ring-opened and oxidized, resulting in a mass shift of 14 Da for each beta-linked sugar. The MALDI–TOF spectra of the peracetylated glycans synthesized by Gtf1/2/3 and DUF1792 before and after oxidation are shown in Fig. 4c,d , respectively. The molecular ion of the oxidized glycan is shifted by 28 Da, which is attributable to two sugars being oxidized, indicating that both of the glucoses are beta-linked. Collectively, the above data demonstrate the functional conservation of DUF1792 as a beta-glucosyltransferase. 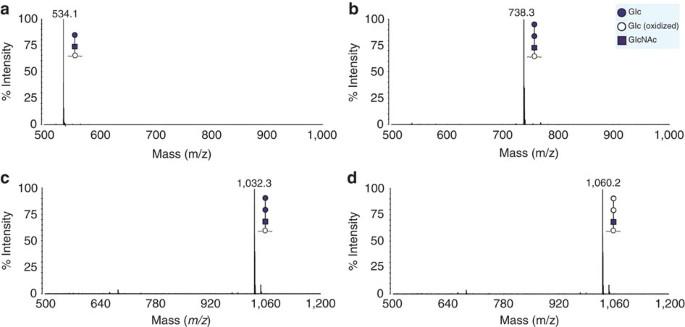Figure 4: MS spectra confirmingin vivoglycosyltransferase activity of DUF1792. The MALDI–TOF spectra of permethylated recombinant Fap1 glycans modified by Gtf1/2/3, and Gtf1/2/3 plus DUF1792 are shown ina,b, respectively. The shift of 204 inm/zcorresponding to a permethylated hexose is consistent with the glucosyltransferase activity of DUF1792. Fap1 glcans modified by Gtf1/2/3 shown inbwere peracetylated and oxidized by CrO3. MALDI–TOF spectra of the trisaccharide from recombinant Fap1 expressed with Gtf1/2/3 and DUF1792, which was analysed as its peracetylated derivative before and after CrO3oxidation, are shown inc,d, respectively. A shift of 28 inm/zcorresponding to two oxidations indicates both linkages are β. Figure 4: MS spectra confirming in vivo glycosyltransferase activity of DUF1792. The MALDI–TOF spectra of permethylated recombinant Fap1 glycans modified by Gtf1/2/3, and Gtf1/2/3 plus DUF1792 are shown in a , b , respectively. The shift of 204 in m/z corresponding to a permethylated hexose is consistent with the glucosyltransferase activity of DUF1792. Fap1 glcans modified by Gtf1/2/3 shown in b were peracetylated and oxidized by CrO 3 . MALDI–TOF spectra of the trisaccharide from recombinant Fap1 expressed with Gtf1/2/3 and DUF1792, which was analysed as its peracetylated derivative before and after CrO 3 oxidation, are shown in c , d , respectively. A shift of 28 in m/z corresponding to two oxidations indicates both linkages are β. Full size image Overall structure of DUF1792 To further characterize this highly conserved new family of glycosyltransferases, we solved the X-ray crystal structure of DUF1792 from S. parasanguinis . The structure of DUF1792 was built by selenomethionyl substituted protein X-ray data utilizing the MAD method ( Table 1 ). Both native protein (Native DUF1792) and the native protein in complex with Mn (DUF1792-Mn) crystallize in a space group of C2 and exist as a monomer. In the native structure, a uridine diphosphate (UDP) molecule and one acetate ion were found ( Supplementary Fig. 3 ). In the DUF1792-Mn structure, a UDP, a manganese and two acetate ions were present ( Fig. 5a,c ). Table 1 Data collection and refinement statistics for DUF1792 from S. parasanguinis . 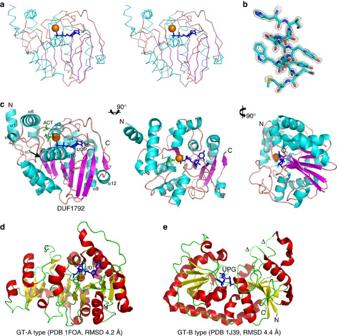Figure 5: The overall structure of DUF1792 (DUF1972-Mn). (a) Stereo image of the backbone trace of DUF1792. The alpha helices are coloured cyan, the beta strands are coloured magenta and coiled regions are salmon and the UDP molecule at the active site is shown in blue and the Mn atom in orange. (b) Representative 2Fo–Fc electron density for DUF1792-Mn. Electron density for the helical region between residue 223-233 is shown in grey and contoured at 2sigma. (c) The overall structure of UDP and Mn-bound DUF1792. The manganese ion is coloured orange, the UDP molecule is blue, beta strands are magenta, alpha helices are cyan and coiled regions are salmon. Two acetate ions are found at the active site and are coloured green. The secondary structural elements are shown in the figure on the left. Three views are shown (left, middle and right). (d) Archetypical GT-A-type glycosyltransferase (PDB id code 1FOA). (e) Archetypical GT-B type glycosyltransferase (PDB id code 1J39). Full size table Figure 5: The overall structure of DUF1792 (DUF1972-Mn). ( a ) Stereo image of the backbone trace of DUF1792. The alpha helices are coloured cyan, the beta strands are coloured magenta and coiled regions are salmon and the UDP molecule at the active site is shown in blue and the Mn atom in orange. ( b ) Representative 2Fo–Fc electron density for DUF1792-Mn. Electron density for the helical region between residue 223-233 is shown in grey and contoured at 2sigma. ( c ) The overall structure of UDP and Mn-bound DUF1792. The manganese ion is coloured orange, the UDP molecule is blue, beta strands are magenta, alpha helices are cyan and coiled regions are salmon. Two acetate ions are found at the active site and are coloured green. The secondary structural elements are shown in the figure on the left. Three views are shown (left, middle and right). ( d ) Archetypical GT-A-type glycosyltransferase (PDB id code 1FOA). ( e ) Archetypical GT-B type glycosyltransferase (PDB id code 1J39). Full size image The structure of DUF1792 consists of 277 residues organized into seven β-strands in the centre, tightly surrounded by 12 α-helices, which appear as a sandwich ( Fig. 5a ). Seven β-strands, β1 (25–29), β2 (67–70), β3 (142–148), β4 (165–171), β5 (195–199), β6 (217–220) and β7 (269–271), form a parallel β-sheet in the topological order β2–β1–β6–β5–β3–β4–β7. The sheet is flanked by eight helices α1 (1–6), α5 (78–80), α6 (83–103), α2 (12–22), α7 (112–115), α8 (126–138), α11 (224–233) and α12 (261–266) on one side, and four helices α3 (31–38), α4 (49–60), α9 (176–191) and α10 (202–214), on the other side. The DUF1792 structure is composed of three regions: the N-terminal region formed from helices α1, α2, α3, α4, α5 and two strands β1 and β2; α 2 β 1 α 3 and α 4 β 2 α 5 form sandwich domains consisting of the metal-binding site, the DXE motif; α 6 and α 7 form a long turn-helix-coil that connects the N-terminal region and the central region. The central region contains a Rossmann-like fold (β 4 α 9 β 5 α 10 β 6 ). The C-terminal region is composed of a long coil region, a short helical turn (α 12 ) and a short β-strand (β 7 ). The nucleotide-binding sites are located at the edge of the β-sheet (β1 and β6), helices α3 and α7 and the C-terminal loop. The DUF1792 structure is distinctly different from the two classic glycosyltransferase folds, GT-A and GT-B ( Fig. 5d,e ). In addition, it does not share any structural similarity with a previously suggested GT-C fold. The DUF1792 structure represents a new GT fold To date, numerous structures have been solved and reported for glycosyltransferases. Structural alignment of DUF1792 performed using the Secondary Structure Matching server [40] from the European Bioinformatics Institute revealed that the closest match is the class B nonspecific acid phosphatase (AphA protein, Protein Data Bank (PDB) entry 1Z5G) from Salmonella typhimurium , with a RMSD deviation of 4.7 Å. AphA has a haloacid dehalogenase-like fold that is conserved in members of the DDDD superfamily of phosphohydrolases [41] . Upon visual inspection, it is clear that only the so-called Rossmann-like fold of the DUF1792 structure superimposes on the haloacid dehalogenase-like structure of AphA ( Fig. 6a ). A general search using the DALI server [42] indicated that the closest match to DUF1792 in the database is 3-Dehydroquinate Synthase (DHQS) from Vibrio cholerae (PDB entry 3OKF) with a weak Z score of 4.8 and a RMS deviation of 3.3 Å ( Fig. 6b ). DHQS catalyses the formation of the first cyclic compound (3-Dehydroquinate) of the shikimate pathway, a promising target for the design of antimicrobial compounds [43] . DHQS requires NAD and a divalent cation to catalyse the reaction [44] . The similarity between DUF1792 and DHQS only extends to the Rossmann-like fold. In addition, there is no sequence homology among the three proteins. Key conserved residues important for glycosyltransferase activity among DUF1792 homologues ( Fig. 3c ) are not found in either DHQS or AphA, further suggesting that DUF1792 represents a new type of glycosyltransferase fold. Despite structures of a large number of glycosyltransferases from two well-defined GT folds being resolved and documented [8] , [9] , [10] , the search failed to identify any structural homologue of DUF1792 from this large pool of reported glycosyltransferases and only revealed a weak homology to two non-glycosyltransferase enzymes, AphA and DHQS, further suggesting that the structure of DUF1792 is unique. As this structure is distinct from two currently defined GT folds, GT-A and GT-B, and a previously designated GT-C fold [15] , [45] , [46] , we have named it as the GT-D fold. 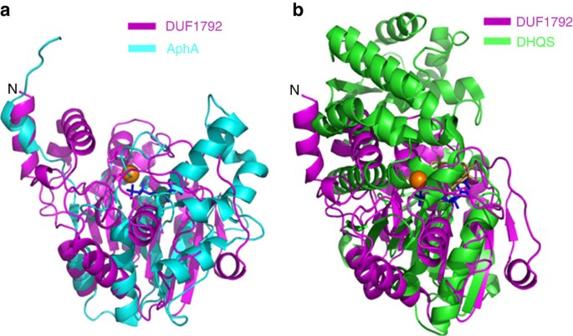Figure 6: Structural alignment of DUF1792. (a) DUF1792 superimposed on molecule A of AphA (PDB id code 1Z5G). DUF1792 is shown in magenta cartoon and AphA is shown in cyan cartoon. (b) DUF1792 superimposed onto molecule A of DHQS (PDB id code 3OKF). DUF1792 is shown in magenta cartoon, and DHQS is shown in green cartoon. The UDP molecule in DUF1792 is shown as blue stick and the Mn ion shown as an orange sphere. The nicotinamide adenine dinucleotide is shown in sand colour stick along with the phosphate ion. Figure 6: Structural alignment of DUF1792. ( a ) DUF1792 superimposed on molecule A of AphA (PDB id code 1Z5G). DUF1792 is shown in magenta cartoon and AphA is shown in cyan cartoon. ( b ) DUF1792 superimposed onto molecule A of DHQS (PDB id code 3OKF). DUF1792 is shown in magenta cartoon, and DHQS is shown in green cartoon. The UDP molecule in DUF1792 is shown as blue stick and the Mn ion shown as an orange sphere. The nicotinamide adenine dinucleotide is shown in sand colour stick along with the phosphate ion. Full size image The GT-D fold possesses UDP and manganese-binding sites The hallmark of glycosyltransferases is their ability to bind to nucleotide-activated sugars [47] . Our biochemical assays revealed that UDP–glucose is the activated sugar used by DUF1792. In fact, during the crystallization of DUF1792, we found UDP–glucose is critical for recombinant DUF1792 to grow crystals. Presumably, the structure of DUF1792 would require the presence of UDP–glucose. However, only UDP was found in the electron-density map from DUF1792 ( Fig. 5a,c and Fig. 7a ), and there was no density for the glucose moiety from UDP–glucose, indicating that the glucose residue may be turned over by in-crystal catalysis. The same phenomenon has been observed for a number of glycosyltransferases using UDP–glucose [36] , [48] or other activated sugar donors [49] , [50] . 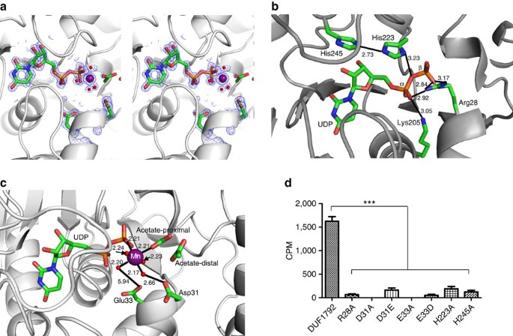Figure 7: DUF1792 possesses UDP and manganese-binding sites. (a) Cross-eyed stereo view showing the electron density of UDP and the manganese ion at the active site. The map shown is a simulated annealing composite omit electron density map calculated in Phenix and contoured at 2.0σ. (b) The UDP-binding site. UDP and the amino-acid residues involved in UDP binding are labelled and atomic distances are shown in Ångstroms. (c) Manganese-binding sites. Manganese and amino-acid residues involved in manganese binding are shown and labelled. The atomic distances are shown in Ångstroms. (d) Critical residues within UDP and metal-binding sites required for glycosyltransferase activity of DUF1792. Site-direct mutagenesis was carried out to mutate critical residues that are involved in binding to UDP and Mn2+, the mutant DUF1792 protein variants were assayed for theirin vitroglycosyltransferase activity. The value obtained from three different experiments represent means±s.e.m.’s. Significant differences were indicated by asterisks (***P<0.001). Figure 7: DUF1792 possesses UDP and manganese-binding sites. ( a ) Cross-eyed stereo view showing the electron density of UDP and the manganese ion at the active site. The map shown is a simulated annealing composite omit electron density map calculated in Phenix and contoured at 2.0σ. ( b ) The UDP-binding site. UDP and the amino-acid residues involved in UDP binding are labelled and atomic distances are shown in Ångstroms. ( c ) Manganese-binding sites. Manganese and amino-acid residues involved in manganese binding are shown and labelled. The atomic distances are shown in Ångstroms. ( d ) Critical residues within UDP and metal-binding sites required for glycosyltransferase activity of DUF1792. Site-direct mutagenesis was carried out to mutate critical residues that are involved in binding to UDP and Mn 2+ , the mutant DUF1792 protein variants were assayed for their in vitro glycosyltransferase activity. The value obtained from three different experiments represent means±s.e.m.’s. Significant differences were indicated by asterisks (*** P <0.001). Full size image In nucleotide sugar-binding sites, the key amino-acid residues with positive charges often interact with phosphate atoms. In DUF1792, the side chain of positively charged Arg28 interacts with both α and β phosphates of UDP at a distance of 2.8 and 2.9 Å, respectively ( Fig. 7b ). In addition, the Lys205 N? atom interacts with the α-phosphate of UDP at a distance of 3.05 Å. The phenyl rings of His245 stack to the pentose sugar ribose of UDP ( Fig. 7b ) and His223 Nδ1 interacts with the O3 atom of the α phosphate (3.2 Å; Fig. 7b ). Similarly, a new epimerase responsible for synthesis of dTDP-L-rhamnose, RmlC, has two Arg residues that interact with the α- and β-phosphates of dTDP-phenol [51] , [52] . The first glycosyltransferase involved in the biosynthesis of mycothiol of Corynebacterium glutamicum , MshA, has three Arg residues involved in the interaction with the phosphoesters of UDP [53] . These residues are crucial for activity of RmlC and MshA. Significantly, Arg28, His223 and His245 are conserved amino-acid residues in DUF1792 homologues from both Gram-positive and Gram-negative bacteria ( Fig. 3c ). When Arg28 was mutated to Ala, the activity of the mutant DUF1792 (Arg28Ala) was completely inhibited. His223Ala and His245Ala mutants also exhibited much lower activity than the native DUF1792 ( Fig. 7d ), demonstrating that Arg28, His223 and His245 are indeed important for UDP binding, and that DUF1792 possesses a UDP-binding motif. The DUF1792 domain is a metal-dependent enzyme that requires bivalent metal ions for its activity ( Fig. 2c ). However, it does not have the typical metal-binding motif, DXD, required for GT-A-type glycosyltransferase [54] , [55] . Instead, a DXE motif is found at residues 31–33, albeit it does not directly interact with the manganese atom in the structure ( Fig. 7c ). In fact, when comparing all DUF1792 homologues from streptococci or even from Gram-negative bacteria, we found that the presence of the DXE motif was invariable and absolutely conserved ( Fig. 3c ). To define the requirement of a DXE motif for glycosyltransferase activity in DUF1792, we performed site-directed mutagenesis and mutated DXE to AXE or DXA. The activity was completely inhibited in these DUF1792 mutants. Furthermore, we mutated DXE to EXE or DXD, and observed a significant reduction in the enzyme activity of each mutant ( Fig. 7d ), demonstrating that even the conserved switch between E and D alters the glycosyltransferase activity of DUF1792. These results further suggest that the DXE motif is critical for the glycosyltransferase activity of DUF1792. Close inspection of the structure revealed that the manganese ion bound at the active site of DUF1792 is octahedrally coordinated by only oxygen atoms: four water molecules, an oxygen atom from the β-phosphate of UDP and one oxygen atom from the acetate ion most proximal to the UDP ( Fig. 7c ). Together, these results demonstrate that DUF1792 contains a metal-binding (DXE) motif in this new family of glycosyltransferases. UDP and metal binding are crucial for in vivo glycosylation of Fap1 To determine the requirement of UDP and metal-binding sites in vivo in S. parasanguinis , we selected one key residue Asp31 engaged in the metal binding, and another one His223 involved in the UDP binding, to carry out site-directed mutagenesis and determined the impact of the mutated dGT1 alleles on biogenesis of Fap1 in S. parasanguinis. D31A, D31E and H223A completely inhibited the production of mature Fap1 as determined by mature Fap1-specific mAbF51 antibody ( Fig. 8a , lanes 5–7). The Fap1 variants generated by the dGT1 site-directed mutants ( Fig. 8b , lanes 5–7) show a similar migration pattern to the Fap1 protein from the dGT1 non-mutant ( Fig. 8b , lane 3) when probed by Fap1-peptide-specific antibody mAbE42, further demonstrating the importance of these two motifs in the glycosylation of Fap1 in vivo . 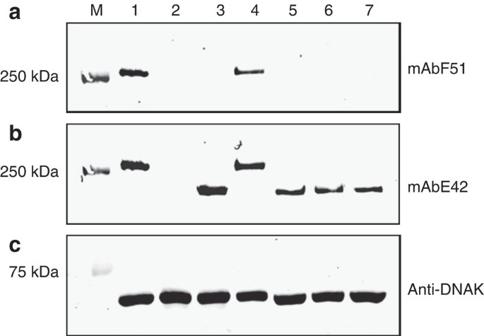Figure 8: UDP and metal binding are required for Fap1 glycosylationin vivo. Wild-type and dGT1 site-directed mutant constructs were used to complement the dGT1mutant inS. parasanguinis. Cell lysates fromS. parasanguinis(1); Fap1 mutant (2); dGT1 mutant (3); the dGT1mutant complemented with the dGT1full-length gene (4), dGT1 (D31A) (5); dGT1(D31E) (6); and dGT1(H223A) (7) were subjected to western blot analysis with Fap1-peptide-specific mAbF51 (a), mature Fap1-specific mAbE42 (b) to determine Fap1 production, and anti-DNAK antibody (c) as a sample loading control. Figure 8: UDP and metal binding are required for Fap1 glycosylation in vivo . Wild-type and dGT1 site-directed mutant constructs were used to complement the d GT1 mutant in S. parasanguinis . Cell lysates from S. parasanguinis (1); Fap1 mutant (2); dGT1 mutant (3); the d GT1 mutant complemented with the d GT1 full-length gene (4), dGT1 (D31A) (5); dGT1(D31E) (6); and dGT1(H223A) (7) were subjected to western blot analysis with Fap1-peptide-specific mAbF51 ( a ), mature Fap1-specific mAbE42 ( b ) to determine Fap1 production, and anti-DNAK antibody ( c ) as a sample loading control. Full size image In this study we have defined a new glycosyltransferase superfamily, DUF1792, which is involved in the biosynthesis of bacterial O-glycans. Glycomic strategies have revealed that Fap1, a bacterial adhesin, is modified by a branched hexasaccharide with the sequence Rha1-3Glcβ1-(Glc1-3GlcNAc1-) 2,6 Glcβ1-6GlcNAc. DUF1792 is a metal-dependent beta-glucosyltransferase, which transfers a Glc residue to the Glc-GlcNAc-modified Fap1 at the branching point. The DUF1792 domain has a Rossmann-like nucleotide-binding fold but does not show any sequence and structure identity with glycosyltransferases possessing currently annotated type GT-A or GT-B folds. The domain does not share any structural identity with a previously proposed GT-C fold either [15] , [45] , [46] . Moreover, DUF1792 has a highly conserved DXE motif instead of the classic DXD metal-binding motif found in the archetypical GT-A folds. Together, our data lead us to propose that DUF1792 represents a new family of glycosyltransferases that display a unique glycosyltransferase fold, which we have named GT-D. The amino-acid sequence constituting the fold is highly conserved in streptococci and even in Gram-negative bacteria. Our biochemical and structural studies of DUF1792 have not only defined the activity of this domain but have also established a new family of bacterial glycosyltransferases with a previously uncharacterized GT fold. This GT-D fold is crucial for Fap1 biogenesis; moreover, the biogenesis of several Fap1-like proteins has been implicated in bacterial virulence [30] . Thus, our characterization of this new GT-D type of glycosyltransferase may be helpful in guiding the design of antibacterial therapeutics targeting this activity. Protein expression and purification The DUF1792 domain encoding amino acids 1–272 of dGT1 (AFJ26875) was amplified from genomic DNA of S. parasanguinis FW213 and cloned into the pET28a-sumo vector and transformed to E. coli BL21 Gold (DE3) cells. All strains and primers used in this study were listed in Supplementary Tables 2 and 3 . The recombinant strain grown to OD 600 =0.8 in LB medium was then induced with 0.1 mM isopropyl-β-D-thiogalactoside at 18 °C overnight. Native DUF1792 protein was purified with Histrap Column (Ni affinity) and gel filtration as described [36] . In brief, the overnight grown E. coli cells were harvested with centrifugation and lysed by sonication in binding buffer (20 mM Tris-HCl pH 8.0, 500 mM NaCl and 25 mM Imidazole). The clear cell lysates obtained after centrifugation (16,500 r.p.m. for 1 h) were subjected to protein purification using HiTrapTM Column (Ni 2+ _affinity). Proteins were eluted from the affinity resin by elution buffer (20 mM Tris-HCl, pH 8.0, 500 mM NaCl and 500 mM imidazole). The N-terminal His-SUMO tag was cleaved by incubating the elution fractions with SUMO protease, ubiquitin-like protein protease, during overnight dialysis at 4 °C against 20 mM Tris-HCl, pH 8.0, 500 mM NaCl. Dialysed protein samples were reapplied to HiTrapTM Column to remove ubiquitin-like protein protease, the cleaved His tag and uncleaved proteins. Flow-through was collected and further purified by using a 16/60 Superdex 75 gel filtration column (GE Healthcare) with gel filtration buffer (20 mM Tris pH 8.0, 100 mM NaCl and 1 mM dithiothreitol (DTT)). Protein purity was analysed using SDS–PAGE. Peak fractions were collected and concentrated to 30 mg ml −l for crystallization screen. Selenomethionyl DUF1792 was obtained by growing the recombinant strain in M9 medium with selenomethionine at 60 mg l −1 (ref. 56 ). The selenomethionyl protein was purified using the same protocol as the native protein. Crystallization, data collection and refinement The purified protein was concentrated to 10 mg ml −l in 20 mM Tris buffer (pH 8.0), 100 mM NaCl, 1 mM DTT and subjected to crystallization trials. Hanging-drop vapour-diffusion method was used for the crystallization trials. Crystals were obtained in the following solution. One microlitre protein solution (10 mg ml −1 ) with 10 mM UDP-Glc was mixed with 1 μl well solution (500 μl) consisting of 100 mM Tris buffer (pH 8.5), 35% PEG 1500, 200 mM Sodium Acetate. A single crystal was cryo-cooled in liquid nitrogen after being cryo-protected by addition of 10% glycerol. The Se-Met-DUF1792 and native DUF1792 in the complex with Mn were crystallized utilizing the same conditions. All DUF1792 crystals appeared in 3 days. Data were collected with an oscillation angle of 1° per image on beamline SER-CAT ID 22 at the Argonne National Laboratory. The structure was determined with multiwavelength anomalous dispersion [15] , utilizing Se atoms as the anomalous scatterers. Se-Met-DUF1792 data were collected at wavelength of 0.97877 (Peak), 0.97907 (Edge) and 0.97142 (High). Data of native DUF1792 and DUF1792-Mn were collected at wavelength of 1,00,000. All data were collected under temperature 100 K. Data were processed and scaled with HKL2000 (ref. 57 ). The model building and subsequent structure refinement were performed with the Phenix software [58] . Restrained individual B-factor and TLS refinement were not performed until the last cycle. After each cycle of refinement, the model was manually rebuilt based on the resulting 2F o –F c and F o –F c maps. Expression and purification of rFap1-RI We used rFap1-RI, a small fragment of Fap1, that contains the first repeat region (100–200 amino-acid residues of Fap1), as a model to carry out glycan profiling study of Fap1. Unglycosylated rFap1-R1 was purified from a recombinant strain that carries pET28a-rFap1-R1. Glycosylated Fap1-R1 was purified from a recombinant BL21 strain that was constructed by co-expression of pET28a-rFap1-R1 with pVPT-Gtf123-dGT1-GalT2 and pHSG576-Gly, in which glycosylated rFap1-R1 was modified by all putative glycosyltransferases, Gtf12, Gtf3, dGT1, GalT2 and Gly. The plasmids and strains were constructed as described in Supplementary Table 2 . All plasmids were confirmed by sequencing. Unglycosylated and glycosylated rFap1-RI were purified using the same method as recombinant DUF1792 protein. Glycan profiling of modified rFap1-R1 Purified rFap1-R1 was subjected to reductive elimination and permethylation as described below. Reductive elimination The glycans were reductively eliminated from rFap1 and purified on a 50E–8C Dowex column as previously described [59] , and the purified glycans were subjected to permethylation and purified according to published methods. Briefly, the freeze-dried rFap1 sample was dissolved in 55 mg ml −1 potassium borohydride in a 1 ml of a 0.1 M potassium hydroxide solution. The mixture was incubated at 45 °C for 18 h and quenched by adding five to six drops of acetic acid. The sample was loaded on the Dowex column and eluted with 5% acetic acid. The collected solution was concentrated and lyophilized. Excessive borates were removed with 10% methanolic acetic acid. Permethylation For the permethylation reaction, sodium hydroxide (three to five pellets per sample) was crushed in 3 ml dry dimethyl sulfoxide. The resulting slurry (0.75 ml) and methyl iodine (500 μl) were added to the sample. The mixture was agitated for 15 min and quenched by adding 2 ml ultrapure water with shaking. The glycans were extracted with chloroform (2 ml) and washed with ultrapure water two times. Chloroform was removed under a stream of nitrogen. The permethylated glycans were loaded on a C18 Sep-pak column, washed with 5 ml ultrapure water and successively eluted with 3 ml each of 15, 35, 50 and 75% aq. acetonitrile. The solutions were collected and lyophilized. Peracetylation A previously described method was used for peracetylation [60] . Glycans were incubated with 200 μl pyridine and 200 μl acetic anhydride at 80 °C for 3 h, after which the reagent was removed under a stream of nitrogen. The acetylated glycans were dissolved in chloroform and washed three times with pure water, and the chloroform was removed under a stream of nitrogen. CrO 3 oxidation CrO 3 (10 mg) was added to 100 μl of acetic acid. The slurry was added to peracetylated samples, and the mixture was heated to 50 °C and kept for 3 h. After quenching the reaction with water, the product of oxidation was extracted with chloroform and washed with water twice. Mass spectrometry MS data were acquired by using either a Voyager DE-STRTM MALDI–TOF or a 4800 MALDI–TOF/TOF mass spectrometer (Applied Biosystems, Darmstadt, Germany). MS/MS data were acquired with the latter instrument. MS mode was calibrated with 4,700 Calibration standard kit (Applied Biosystems), and MS/MS mode was calibrated with fibrinopeptide B human (Sigma). For MS/MS studies, the collision energy was set to 1 kV, and the collision gas was argon. 2, 5-dihydroxybenzoic acid was used as matrix. Permethylated samples were dissolved in 10 μl methanol, 1 μl of this solution was premixed with 1 μl matrix and 1 μl of the mixture was spotted on the plate. GC–MS Trimethylsilyl analysis The glycan sample was incubated with 1.0 M methanolic HCl at 80 °C for 14 h. The reagent was removed under a stream of nitrogen. Methanol (500 μl), pyridine (10 μl) and acetic anhydride (50 μl) were successively added to the sample. The mixture was kept at room temperature for 15 min and the reagent was removed under a stream of nitrogen. Tri-Sil Z reagent (200 μl) was added to the sample, and the mixture was kept at room temperature for 15 min. After removing the reagent under a stream of nitrogen, the sample was washed by hexane twice. A PerkinElmer Clarus 500 instrument fitted with a RTX-5-fused silica capillary column was used for carrying out the analysis. The following temperature programme was used for eluting the sample. The oven temperature was initially 65 °C, and heated to 140 °C at the rate of 25 °C per min, and heated to 200 °C at the rate of 5 °C min −1 . The temperature was finally raised to 300 °C at a rate of 10 °C min −1 and is held for 5 min. GC–MS linkage analysis Partially, methylated alditol acetates were prepared as previously described [61] . A PerkinElmer Clarus 500 instrument fitted with a RTX-5-fused silica capillary column was used for carrying out linkage analysis. A linear gradient temperature programme was used: the sample was injected into the column at 60 °C, and the temperature increases to 300 °C over 30 min at a rate of 8 °C min −1 . Construct of a d gT1 knockout mutant A non-polar d gT1 knockout mutant was generated by insertional mutagenesis with a kanamycin resistance cassette (Kan r ). Briefly, the d gT1 gene and its flanking regions including the 600-bp upstream and 600-bp downstream regions were amplified from genomic DNA of S. parasanguinis FW213. The PCR fragment was purified and cloned into pGEM-T Easy vector (Promega, Madison, WI, USA). A 1,500-bp d gT1 internal fragment was replaced with an 830-bp nonpolar kanamycin resistance cassette ( aphA3 ) isolated from pALH124 (ref. 62 ) by an inverse PCR strategy. Plasmid was confirmed by sequencing and then transformed into the FW213 strain by electroporation. The transformants were selected on TH agar plates containing kanamycin. The d gT1 allelic replacement mutant was selected by its ability to resist kanamycin and its susceptibility to tetracycline and was further verified by PCR and sequencing analysis. The confirmed d GT1 allelic replacement mutant was used in this study. Western blot analysis For all S. parasanguinis strains, bacteria grown to an optical density at 470 nm (OD470) of 0.5–0.6 were harvested using centrifugation. The cell pellets were treated with amidase to lyse the cells [31] . For E. coli strains, bacteria grown to an optical density at 600 nm (OD600) of 0.6–0.7 were harvested by centrifugation. Cell lysates were prepared by boiling the cell pallets collected in sample buffer (0.0625 M Tris-HCl (pH 6.8), 2% sodium dodecyl sulphate (SDS), 10% glycerol, 0.01% bromophenol blue) for 10 min before being loaded onto 8% SDS–polyacrylamide gel electrophoresis (PAGE) gels and subjected to western blotting. Two monoclonal anti-mouse antibodies (MAbs) were used to detect Fap1: MAbE42 (1:3,000), which is specific to the peptide backbone of Fap1, and MAb F51(1:5,000), which is specific to mature Fap1 (ref. 63 ). A polyclonal anti-rabbit antibody against DNAK (a gift from José Lemos at the University of Rochester) was used to standardize the protein loading of S. parasanguinis lysates. All western blot figures shown in this paper were cropped. Uncropped figures are supplied in Supplementary Fig. 4 . Site-direct mutagenesis, in vitro and in vivo Fap1 glycosylation Site-direct mutagenesis was carried out using QuickChange mutagenesis kit (Stratagene) as described [36] . The plasmid pET28a-sumo-DUF1792 and pVPT-dGT1 were used as templates. Mutant constructs were identified and confirmed by sequencing. Mutated DUF1792 proteins were purified using the same method as described above. Gtf1/2, 3-modified rFap1 was purified using Glutathione-Sepharose 4B beads according to the manufacturer’s protocol (Amersham) and used as a substrate for the in vitro glycosyltransferase assays as described previously [35] . In brief, the substrate and enzyme bound to glutathione-Sepharose beads were washed five times with glycosylation buffer (50 mM Hepes, pH 7.0, 10 mM MnCl 2 , 0.01% bovine serum albumin). Recombinant dGT1 (20 μg) or its variants and substrate Fap1 were mixed with 0.2 μCi of UDP-[3H]glucose (28 Ci mmol −1 ; Amersham Biosciences) or 0.2 μCi of UDP-[3H]GlcNAc (2.8 Ci mmol −1 ; Amersham Biosciences) in a final volume of 200 μl of glycosylation buffer and incubated for 1 h at 37 °C. The beads in the glycosylation assays were washed three times with NETN buffer (20 mM Tris-HCl, 100 mM NaCl, 1 mM EDTA, 0.2% NP40, pH 7.0) and then transferred to scintillation vials to measure radioactivity transferred to the Fap1 substrates from the radiolabelled activated sugars. The assays were performed in triplicate in three independent experiments. DUF1792 homologues from S. agalactiae J48, S. pneumonia TIGR4, S. sanguinis SK36 and Fusobacterium nucleatum were amplified from each strain and cloned to pGEX-6p-1 to generate pGEX-DUF1792, respectively. pHSG576-rFap1 (pAL80), pVPT-gtf1-2-3 and pGEX-DUF1792 were co-transformed into E. coli . The ability of DUF1792 homologues to glycosylate Gtf1/2, 3-modified rFap1 was examined using western blotting analysis with Fap1-peptide-specific monoclonal antibody E42 at 1:3,000 dilution. The construct pVPT- dGT1 , pVPT- DUF1792, pVPT- dGT1-Cterminus and site-directed mutants of dGT1 variants were used to transform the d GT1 knockout to determine the effect of site-directed mutations within this DUF1792 domain on Fap1 glycosylation in vivo. Biogenesis of Fap1 was detected by western blotting analysis using the Fap1-specific monoclonal antibodies E42 (peptide-specific) and F51 (mature Fap1). Statistics The two-tailed Student’s t -test was used to determine statistically significant differences between groups and statistically significant differences with P values below 0.006 are indicated with two asterisks (**) and below 0.0006 are indicated with three asterisks (***). Accession codes: Coordinates and structure factors for DUF1792-Mn, DUF1792-native and DUF1792 (Se-Met) crystal structures have been deposited in the Protein Data Bank with the succession numbers 4PHR , 4PFX and 4PHS respectively. How to cite this article: Zhang, H. et al. The highly conserved domain of unknown function 1792 has a distinct glycosyltransferase fold. Nat. Commun. 5:4339 doi: 10.1038/ncomms5339 (2014).